Microwave cavity-enhanced transduction for plug and play nanomechanics at room temperature Following recent insights into energy storage and loss mechanisms in nanoelectromechanical systems (NEMS), nanomechanical resonators with increasingly high quality factors are possible. Consequently, efficient, non-dissipative transduction schemes are required to avoid the dominating influence of coupling losses. Here we present an integrated NEMS transducer based on a microwave cavity dielectrically coupled to an array of doubly clamped pre-stressed silicon nitride beam resonators. This cavity-enhanced detection scheme allows resolving of the resonators' Brownian motion at room temperature while preserving their high mechanical quality factor of 290,000 at 6.6 MHz. Furthermore, our approach constitutes an 'opto'-mechanical system in which backaction effects of the microwave field are employed to alter the effective damping of the resonators. In particular, cavity-pumped self-oscillation yields a linewidth of only 5 Hz. Thereby, an adjustement-free, all-integrated and self-driven nanoelectromechanical resonator array interfaced by just two microwave connectors is realised, which is potentially useful for applications in sensing and signal processing. The increasing importance of nanomechanical resonators for both fundamental experiments [1] , [2] , [3] and sensing applications [4] , [5] in recent years is a direct consequence of their high resonance frequencies as well as low masses. However, because of their small size, they couple only weakly to their environment, which can make it difficult to efficiently transduce their motion. This coupling can be strongly enhanced via an optical [6] , [7] , [8] , [9] , [10] , [11] or electrical microwave [12] , [13] , [14] , [15] , [16] , [17] cavity. While both methods enable sensitive displacement detection, only the latter is suitable for large-scale integration of many resonators with a single cavity. Up to now, nanoelectromechanical transduction via microwave cavities is predominantly performed at cryogenic temperatures to benefit from superconducting cavities capacitively coupled to superconducting mechanical resonators. With a main focus on quantum mechanical ground state cooling [2] , the potential of cavity nanoelectromechanical systems (NEMS) for integrated transduction at room temperature is yet to be exploited. To this end, we present an approach based on a copper microstrip cavity operating at 300 K. While previous works [12] , [13] , [14] , [15] , [16] relied on capacitive coupling between cavity and metallized resonator, we employ a dielectric resonator made of highly stressed silicon nitride. This avoids additional damping by losses in the metallization layer, which frequently is one of the dominating sources of dissipation at room temperature [18] , [19] . For transduction, we take advantage of dielectric gradient forces, which are becoming more and more established as a powerful tool to control NEMS [20] , [21] , [22] , [23] : if a dielectric beam is placed in between two vertically offset electrodes, its vibration will induce a periodic modulation of their mutual capacitance. We demonstrate that this modulation alters the response of a connected microwave cavity, which can be demodulated to probe the displacement of the nanomechanical resonator. The resulting heterodyne cavity-enhanced detection scheme allows probing of the resonator's Brownian motion with a sensitivity of presently at 300 K. We have tested the scheme to operate at temperatures between 300 K and low temperatures (4 K), at which superconducting cavities become superior. Furthermore, the coupled cavity-resonator device is a microwave analogy of an optomechanical system: cavity electromechanics can be employed to amplify or damp the mechanical vibration utilizing the dynamical backaction of the microwave field. By strongly amplifying the motion, the regime of cavity-pumped self-oscillation is reached. The resulting high-amplitude, narrow-band signal with a linewidth of only 5 Hz can be used to track the resonance frequency of the beam, yielding an estimated mass resolution of about 10 −18 g. Device and measurement setup Arrays of mechanical beam resonators of different length are fabricated out of a 100-nm-thick pre-stressed silicon nitride film deposited on a fused silica wafer (see Fig. 1a for one element as well as Methods and Supplementary Fig. S1 ). Each nanomechanical resonator is embedded in a capacitive structure, which is part of the resonant LC circuit as sketched in Fig. 1a,b and c,d , respectively. One of the electrodes is connected to an external λ /4 microstrip cavity (see Fig. 1d and Methods) with a resonance frequency of f c =3.44 GHz and a quality factor of 70, the transmission of which is shown in Fig. 1c . In contrast to the more common SiN films on silicon substrates, SiN on fused silica avoids room temperature dissipation of microwave signals by mobile charge carriers and generates an even higher tensile stress in the SiN film [24] . Measuring the resonance frequencies of several harmonic modes and fitting these with a simple theoretical model [25] yields a beam stress of 1.46±0.03 GPa. Recently, it has been demonstrated that the tensile stress in a nanomechanical resonator enhances its eigenfrequency and quality factor [25] , [26] . Thus, the observed quality factors are higher than the ones measured with resonators of the same eigenfrequency on a silicon substrate with a prestress of 0.83 GPa, and beams of the same length have higher resonance frequencies. Whereas the described scheme has been employed on a range of microwave cavities and nanomechanical resonator arrays, all measurements shown here have been performed on one 55 μm long beam with a fundamental mechanical resonance frequency of f m =6.6 MHz and a room temperature quality factor Q m =290,000. 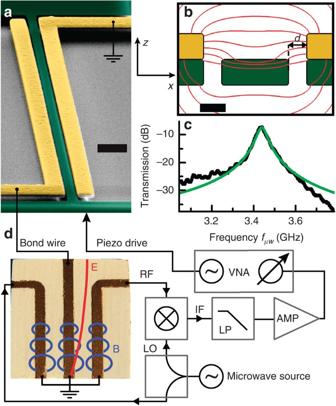Figure 1: Sample and setup. ashows a scanning electron micrograph of the 55 μm long silicon nitride beam (green) flanked by two gold electrodes (yellow). Scale bar corresponds to 1 μm. The schematic cross-section of the beam and electrodes inb(scale bar corresponds to 100 nm) exhibits a symmetric gap ofd=60 nm and includes simulated electric field lines. The beam is placed just below the electrodes, where its movement in thezdirection induces the largest modulation of the capacitance. The electrodes are connected to an electrical λ/4 microwave cavity via bond wires.cdepicts its transmission spectrum (black) with a Lorentzian fit (green). The schematic circuit diagram shown indincludes a photo of the cavity circuit board (8×8 mm2). It also illustrates magnetic field lines (blue) indicating the inductive coupling between the two side electrodes and the central resonator, and the electric field distribution (red) in the resonator. The cavity is pumped by a microwave source, the radio frequency transmission signal is mixed with a reference signal (LO) such that the mechanical sidebands (IF) are demodulated. A lowpass filter (LP) is used to remove higher-frequency components, and the amplified (AMP) sideband signal is fed to a vector network analyser (VNA), which can also drive a piezo to actuate the beam. See Fig. 5 and Methods for the detailed circuit. Figure 1: Sample and setup. a shows a scanning electron micrograph of the 55 μm long silicon nitride beam (green) flanked by two gold electrodes (yellow). Scale bar corresponds to 1 μm. The schematic cross-section of the beam and electrodes in b (scale bar corresponds to 100 nm) exhibits a symmetric gap of d =60 nm and includes simulated electric field lines. The beam is placed just below the electrodes, where its movement in the z direction induces the largest modulation of the capacitance. The electrodes are connected to an electrical λ/4 microwave cavity via bond wires. c depicts its transmission spectrum (black) with a Lorentzian fit (green). The schematic circuit diagram shown in d includes a photo of the cavity circuit board (8×8 mm 2 ). It also illustrates magnetic field lines (blue) indicating the inductive coupling between the two side electrodes and the central resonator, and the electric field distribution (red) in the resonator. The cavity is pumped by a microwave source, the radio frequency transmission signal is mixed with a reference signal (LO) such that the mechanical sidebands (IF) are demodulated. A lowpass filter (LP) is used to remove higher-frequency components, and the amplified (AMP) sideband signal is fed to a vector network analyser (VNA), which can also drive a piezo to actuate the beam. See Fig. 5 and Methods for the detailed circuit. Full size image By coupling the mechanical resonator to the microwave cavity, the electrical resonance frequency f c is periodically modulated, causing sidebands at f c ± f m in the microwave transmission signal. These are demodulated, filtered and amplified (see Fig. 1d , Fig. 5 and Methods), then fed directly into a vector network analyser, the output of which can be used to excite the mechanical resonator via a piezo inertial drive [26] . The resonator chip, glued onto the piezo transducer, as well as the cavity are operated in a vacuum chamber at pressures below 5×10 −4 mbar at room temperature. Detection The amplitude of the piezo-driven mechanical resonator ( Fig. 2a ) is probed by monitoring the sideband signal via the demodulated microwave transmission signal. Note that all amplitudes in this work are given as half-peak-to-peak values. A Lorentzian fit is used to extract the mechanical resonance amplitude, which depends on the output power P μw and frequency f μw of the microwave source. 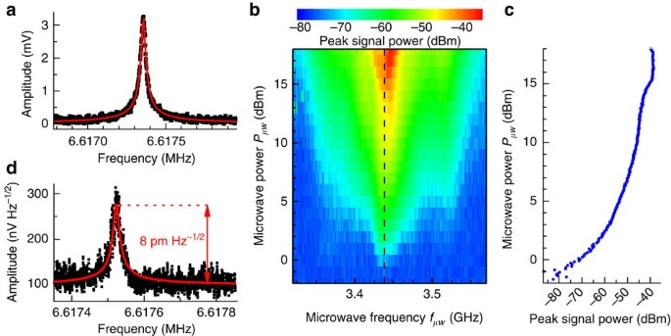Figure 2: Detection. The driven response of the 55 μm long beam is shown ina. It is vibrating with an amplitude of about 6 nm at a piezo-driving power of −70 dBm measured with a microwave power ofPμw=18 dBm atfμw=3.44 GHz. To determine the operating regime of the detection scheme as a function of the cavity parameters, microwave frequency and power are systematically varied and the mechanical peak signal power reflecting the squared resonance amplitude (that is, the maximum of the resonance ina) is plotted inbfor each point. A cut along the microwave cavity resonance (dashed line inb) shown incdepicts that the detected signal is maximized at cavity powers between 15 and 18 dBm. The Brownian motion of the resonator indis employed to deduce the sensitivity of the detection scheme from the noise floor. Figure 2b shows how the operating range of the detection mechanism can be mapped out by systematically varying the microwave parameters. The plot displays the colour-coded peak signal power of the mechanical spectrum, plotted for every set of P μw and f μw . Maximum sensitivity is achieved on resonance with the microwave cavity (at f μw = f c =3.44 GHz, dashed line), where the cavity field and its sensitivity to frequency changes are maximized. The peak signal power in Fig. 2c is directly proportional to the microwave power at low levels, but nonlinear effects in the cavity cause the detection efficiency to level off above P μw =15 dBm. Using the optimal operating point of f μw = f c and P μw =18 dBm, the thermally induced Brownian motion of the resonator can be easily resolved, as depicted in Fig. 2d . By calculating the thermal amplitude of the beam to be at room temperature, the observed noise level corresponds to a sensitivity of (see also Supplementary Methods ). Thus, the full dynamic range of the resonator is accessible as the detection scheme allows to characterize the resonator response from the thermal motion until the onset of nonlinear behaviour. Figure 2: Detection. The driven response of the 55 μm long beam is shown in a . It is vibrating with an amplitude of about 6 nm at a piezo-driving power of −70 dBm measured with a microwave power of P μw =18 dBm at f μw =3.44 GHz. To determine the operating regime of the detection scheme as a function of the cavity parameters, microwave frequency and power are systematically varied and the mechanical peak signal power reflecting the squared resonance amplitude (that is, the maximum of the resonance in a ) is plotted in b for each point. A cut along the microwave cavity resonance (dashed line in b ) shown in c depicts that the detected signal is maximized at cavity powers between 15 and 18 dBm. The Brownian motion of the resonator in d is employed to deduce the sensitivity of the detection scheme from the noise floor. Full size image As the detected signal is only proportional to the change in capacitance dC / dz caused by a displacement dz and other geometrical parameters, the displacement sensitivity is independent of the mechanical frequency. However, higher-frequency beams imply a reduced electrode length and thus weaker coupling for constant cross-section of the detection capacitor. The same applies to higher harmonic modes, where only one antinode of odd harmonic modes generates a signal, as the other antinodes cancel each other. This results in a 1/ f scaling of the sensitivity in the case of a stressed string, as observed in other measurements for beams with frequencies between 6 and 60 MHz. Furthermore, even the in-plane motion of the beam can be detected (not shown). Considering the electrode geometry displayed in Fig. 1b , this seems to be suprising at first. Ideally, the capacitance gradient dC / dx is a parabola such that both a displacement of the beam in positive and negative x direction increases the capacitance symmetrically. Thus, there should be no signal on the resonance frequency of the mode. But even small imperfections during sample fabrication lead to a slightly off-centre position of the beam and thereby a non-zero capacitance gradient in the x direction. Therefore, in-plane modes are accessible, albeit with a lower sensitivity such that the Brownian motion cannot be resolved. Backaction effects For a detuned microwave cavity, the coupling between the cavity and the mechanical resonator gives rise to 'opto'-mechanical effects such as backaction cooling and pumping of the mechanical mode [2] , [3] , [6] , [7] , [8] , [9] , [10] , [11] , [12] , [16] , [17] , [27] , [28] . The signature of these cavity electromechanical effects can already be discerned in the red portion of Fig. 2b and is shown more clearly in Fig. 3 . Comparison of the different mechanical resonance curves obtained for negative, positive and no detuning (inset of Fig. 3a ) shows that both the resonance amplitudes ( Fig. 3a ) and the measured, effective Q (Δ) ( Fig. 3b , see Supplementary Methods ) change with detuning. If the detuning Δ= f μw − f c between microwave drive and cavity resonance frequency is negative (red detuned), the electrical force produced by the cavity field counteracts the vibrational motion, thereby decreasing its amplitude. For positive (blue) detuning, the amplitude is increased. As the resonance amplitude depicted in Fig. 3a is superimposed with the detuning-dependent sensitivity curve discussed in Fig. 2b and therefore distorted, we rather use the detuning dependence of the quality factor to analyse the data. 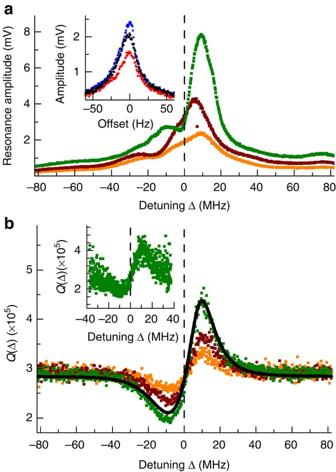Figure 3: Cavity electromechanics. Resonance amplitude and quality factor of the weakly driven (piezo power of −70 dBm) mechanical mode are increased or decreased depending on the microwave detuning Δ=fμw−fcdue to the backaction of the microwave field on the resonator. This is shown in the inset ofa, comparing resonance curves of the same resonance at a microwave power of 12 dBm for red, blue or no (red, blue and black points, respectively) detuning. For clarity, the resonance curves have been plotted versus the frequency offset to the respective (detuning-dependent) resonance frequency. Panelashows the detuning dependence of the resonance amplitude (that is, maximum in inset) for different microwave powers of 18, 15 and 12 dBm (green, red and orange dots). Inb, the detuning dependence of the quality factor for the same power values is depicted, along with a fit to the theoretical model (black line, seeSupplementary Methods). The inset ofbshows the quality factor of the Brownian motion versus detuning at 18 dBm microwave power with identical axes, the only difference to the main plot is the better signal to noise ratio in the weakly driven case. Figure 3: Cavity electromechanics. Resonance amplitude and quality factor of the weakly driven (piezo power of −70 dBm) mechanical mode are increased or decreased depending on the microwave detuning Δ= f μw − f c due to the backaction of the microwave field on the resonator. This is shown in the inset of a , comparing resonance curves of the same resonance at a microwave power of 12 dBm for red, blue or no (red, blue and black points, respectively) detuning. For clarity, the resonance curves have been plotted versus the frequency offset to the respective (detuning-dependent) resonance frequency. Panel a shows the detuning dependence of the resonance amplitude (that is, maximum in inset) for different microwave powers of 18, 15 and 12 dBm (green, red and orange dots). In b , the detuning dependence of the quality factor for the same power values is depicted, along with a fit to the theoretical model (black line, see Supplementary Methods ). The inset of b shows the quality factor of the Brownian motion versus detuning at 18 dBm microwave power with identical axes, the only difference to the main plot is the better signal to noise ratio in the weakly driven case. Full size image The effective Q (Δ) in Fig. 3b clearly shows the expected behaviour: at negative detuning, the additional cavity-induced damping Γ(Δ) is positive, such that the effective damping exceeds the intrinsic value and Q (Δ) decreases, whereas at positive detuning the opposite occurs, with an optimal detuning of |Δ opt |=9 MHz. Fitting the theoretical model (refs 27 , 28 , 29 and Supplementary Methods ) to the data measured at several cavity drive powers allows to extract the average coupling factor . The backaction effect is independent of piezo-driven beam actuation as only the effective damping is changed. This is confirmed by repeating the experiment without piezo actuation (inset of Fig. 3b ). A comparison between the weakly driven situation depicted in Fig. 3b and the Brownian motion in the inset only shows a significant increase of the noise in the latter case. Therefore, all measurements in Figs 3 and 4a (except the inset in Fig. 3b ) were done with a weak piezo actuation of −70 dBm to operate with an improved signal to noise ratio. 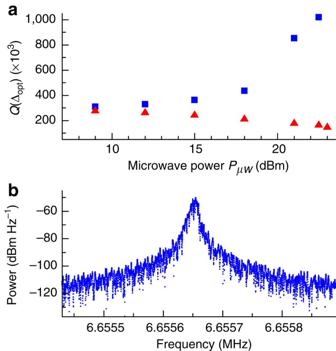Figure 4: Cavity-induced damping and self-oscillation. Using a blue-detuned (red-detuned) cavity drive, the amplitude of the beam can be amplified (damped). This effect is controlled by the microwave powerPμw, as shown ina(blue squares: blue detuning, red triangles: red detuning) for the optimal Δoptof ±9 MHz. By increasing the microwave power to 23 dBm, the backaction gain caused by the blue-detuned cavity exceeds the intrinsic damping, and self-oscillation occurs. The respective power spectrum inbshows a linewidth reduced to 5 Hz. Figure 4: Cavity-induced damping and self-oscillation. Using a blue-detuned (red-detuned) cavity drive, the amplitude of the beam can be amplified (damped). This effect is controlled by the microwave power P μw , as shown in a (blue squares: blue detuning, red triangles: red detuning) for the optimal Δ opt of ±9 MHz. By increasing the microwave power to 23 dBm, the backaction gain caused by the blue-detuned cavity exceeds the intrinsic damping, and self-oscillation occurs. The respective power spectrum in b shows a linewidth reduced to 5 Hz. Full size image Increasing the microwave power to 23 dBm, the quality factor can be decreased to half its initial value with a negative Δ as shown in Fig. 4a , corresponding to an effective mode temperature of 150 K (ref. 6 ). For positive Δ, the quality factor diverges. This reflects cavity-driven self-oscillation of the beam, once the intrinsic damping is cancelled by the cavity backaction. The power spectrum of this oscillation is shown in Fig. 4b . Its linewidth of 5 Hz, corresponding to an effective quality factor [30] of 1.3 million, is limited by the stability of the oscillation frequency, which is mainly affected by fluctuations of the cavity drive. This ultra-low linewidth is ideally suited for mass-sensing applications, giving rise to an estimated mass resolution of about 10 −18 g (see Supplementary Methods ). In contrast to single carbon nanotubes, which have been employed to probe masses of 10 −22 g (refs 4 , 5 ), the presented scheme can readily be scaled up to a large-scale fabrication process involving many beams. Further improvements can be expected by increasing the electromechanical coupling constant [2] , [13] . This can be achieved by a reduced gap size in the detection capacitor. Beam–electrode separations of 20 nm have already been demonstrated [15] , which should yield a tenfold increase in coupling. Besides the backaction effects, there is a quasistatic electric force acting on the resonator [21] . The electric microwave field between the electrodes polarizes the dielectric beam, creating dipoles that are attracted to high electric fields. This leads to an additional effective spring constant that scales with the square of the field (that is, with P μw ) and leads to an increased (decreased) restoring force for the out-of-plane (in-plane) mode. The resulting difference in resonance frequency is clearly visible comparing Fig. 2a ( P μw =18 dBm) to Fig. 4b ( P μw =23 dBm) and can be employed to tune the mechanical eigenfrequency. There are only a few existing nanomechanical transduction schemes at room temperature providing good integration and scalability to large resonator arrays coupled to a single readout cavity: photonic circuits [31] , [32] , [33] offer extremely large displacement sensitivities, but are limited by the precise alignment of external components and thus sensitive to vibrations. On the other hand, adjustment-free schemes such as piezoelectric transduction [34] or capacitive detection [13] , [35] , which, in addition, frequently require cryogenics, impose material constraints and can cause additional dissipation [18] , [19] . In contrast, the presented dielectric coupling of the nanomechanical resonator to the microwave cavity allows to maintain a large quality factor over a wide temperature range (tested between 4 and 300 K). Accordingly, the reported room temperature Q m of 290,000 of the prestressed SiN-on-fused-silica nanoresonator is, to our knowledge, the highest ever obtained in this frequency range. In conclusion, we present a room temperature platform for the sensitive readout, actuation and tuning of nanomechanical resonators. We achieve a sensitivity well below the Brownian motion for the fully integrable and robust heterodyne readout of a nanomechanical resonator via a weakly coupled microwave cavity . This coupling constant is significantly smaller than the one obtained with capacitively coupled beams [13] but requires neither cryogenics nor beam metallization. The relative cavity frequency shift g / f c is comparable to typical optical experiments [22] , [36] , as not only the coupling constant g but also the cavity resonance frequency f c are orders of magnitude smaller in the microwave regime. A major advantage of the presented scheme is the parallel readout of many beams and many modes (higher harmonics as well as in- and out-of-plane) using only a single microwave setup. Additionally, the cavity backaction can be used to control the amplitude of the resonator, thus allowing to omit the piezo actuator. By entering the regime of cavity-pumped self-oscillation a strong and narrow-band signal is generated, perfectly suited for sensing applications requiring a simple resonance frequency readout. As both resonator and cavity are fabricated reproducibly using standard lithographic processes, inexpensive plug and play NEMS sensor modules using only two microwave connectors to interface them with control electronics can be developed. Microwave setup The microwave cavity is fabricated on a ceramic substrate suitable for high-frequency applications (Rogers TMM10) cut to small chips. Standard optical lithography and wet etch processes are employed to pattern the 17 μm thick top copper layer, onto which a 150 nm gold coating is evaporated to avoid corrosion. The design of the microwave cavity shown in Fig. 1d consists of an 8 mm long and 0.64 mm wide centre strip that forms the actual λ/4 resonator. One end of the strip is grounded, while its other end is connected to the silica chip carrying the mechanical resonators. Two adjacent strips near the grounded end are used to inductively couple the cavity to the feed lines and measure the transmission signal. We chose inductive coupling to separate the interface to the chip at the open end from the interface to the feed lines at the grounded end of the λ/4 resonator. The length of the two feed lines (6 mm) and the distance between the striplines (1.2 mm) were optimized using high-frequency circuit simulations with APLAC for a tradeoff between transmission and quality factor of the cavity. 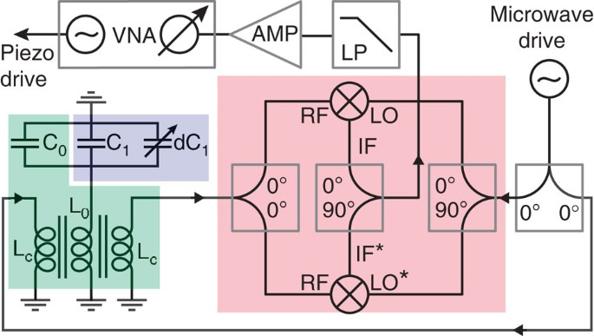Figure 5: Detailed electrical schematic. Detailed version ofFig. 1dshowing an electrical equivalent circuit of the microwave cavity (green box) coupled to the resonator chip (blue box) and the complete IQ mixing circuit (red box). The two signal paths offset by 90° are denoted LO/IF and LO*/IF*, respectively. Figure 5 shows a detailed version of the simplified electrical circuit depicted in Fig. 1d . On the left, the electrical equivalent circuit of the λ/4 microstrip cavity including both feed lines and the coupling to the chip is depicted. The actual cavity consists of the inductance L 0 of the 8 mm long copper strip and its capacitance C 0 to the ground plane on the bottom of the circuit board. The inductive coupling between L 0 and the two feed lines with inductances L c provides the external interface to the cavity. The resonator chip is connected to the open end of the cavity, it adds a static capacitance C 1 and a time-dependent contribution d C 1 ( t ), which oscillates with the actual beam displacement. A very rough estimate for L 0 and C 0 can be obtained from microstrip theory, giving values of 1 pF and 3 μH (this would result in ), neglecting the effects of the microstrip ends. As the resonance frequency of the bare microwave cavity is about 5% higher than with the bond wire and chip connected, C 1 must be <10% of C 0 , as the bond wire also adds some inductance to the circuit. Figure 5: Detailed electrical schematic. Detailed version of Fig. 1d showing an electrical equivalent circuit of the microwave cavity (green box) coupled to the resonator chip (blue box) and the complete IQ mixing circuit (red box). The two signal paths offset by 90° are denoted LO/IF and LO*/IF*, respectively. Full size image A microwave tone is applied to one port of the cavity, thus creating a phase-modulated signal at the other port of the cavity caused by the alternating capacitance d C 1 . As the transmission through the cavity also adds some detuning-dependent phase to the microwave tone, directly mixing the cavity output with the drive tone would result in a detuning-dependent phase difference between the two signals. This difference would need to be compensated for by an additional phase shifter, which had to be adjusted for maximum signal at every drive frequency. To avoid this tedious procedure, we use an IQ (in-phase/quadrature) mixer shown in the red box in Fig. 5 . It consists of a 0°/0° and a 0°/90° power splitter as well as two mixers. The reference signal coming from the microwave generator is split into two parts with a 90° phase shift to each other. By mixing these two signals (LO and LO*) with the radio frequency transmission signal of the cavity, two intermediate frequency signals (IF and IF*) are created. Depending on the phase of the two input signals of the IQ mixer, at least one of these signals is always non-zero, and their (phase-correct) sum is completely independent of the phase relation of the input signals. Thus, by combining the two demodulated quadrature components with another 0°/90° power splitter and blocking the higher-frequency mixing products, amplitude and phase of the mechanical signal are reconstructed. The noise background of this signal is primarily caused by the phase noise of the frequency generator driving the electrical cavity, causing more background noise with increasing power. Therefore, we use a Rohde and Schwarz SMA100A signal generator with extremely low phase noise below −150 dBc at 10 MHz offset. In order to preserve the low noise level, the demodulated sidebands are amplified with a 35 dB preamplifier with a noise figure of 1.3 dB. The output of this amplifier is either directly connected to a spectrum analyser (to quantify the Brownian motion) or amplified by another 30 dB and fed to a network analyser (in case of the driven measurements). Resonator fabrication The samples are fabricated on 500 μm thick fused silica wafers, which are coated with a 100 nm thick commercial high-quality LPCVD layer of pre-stressed silicon nitride. Large chips of size 5×5 mm 2 are cut from the wafer. To enable electron beam lithography on these non-conductive substrates, 2 nm of chromium is evaporated onto the PMMA resist before exposure and removed before developing. E-beam lithography and standard lift-off processes are used to define the gold electrodes and a thin cobalt etch mask protecting the beams. The subsequent inductively coupled plasma reactive ion etch using SF 6 and Ar removes the silicon nitride which is not protected by a metal layer. The final hydrofluoric acid wet etch removes the cobalt and releases the beams, while the gold electrodes use chromium as an adhesion layer and are not attacked by the acid. Finally, the chips are blow-dried with nitrogen, glued to the piezo and a wire bonder is used to connect them to the microwave cavity. All these processing steps use industry-standard techniques, so a large-scale fabrication of inexpensive sensor modules should be within reach. Each mechanical resonator chip contains multiple beams with their respective electrodes, all shunted between two bond pads that are used to connect the chip to the microwave cavity. One design with big variations in the beam length is shown in Supplementary Fig. S1 . It is also possible to use designs with very small length differences in the order of 100 nm, allowing to address many mechanical resonances by frequency division multiplexing in a narrow frequency band. Resonator chip design In order to choose the sample design with the highest coupling between the electrical cavity and the mechanical resonator, several simulations of the electrode configuration using COMSOL Multiphysics were conducted. The electrodes were patterned directly onto the SiN film to induce a maximal capacitance variation with beam displacement. We decided to put the gold electrodes on top of the silicon nitride layer and thereby deposit them before the reactive ion etch step, in contrast to our earlier designs where the gold was evaporated onto the remaining silicon dioxide covering the silicon substrate below the resonator [21] . In these previous designs, the vertical separation between the beam and the silicon dioxide layer had to exceed 250 nm to achieve sufficient underetching of the beam. Thus the new design allows for much smaller overall beam–electrode separations, resulting in a larger effect of the beam motion on the capacitance. Further simulations with this principal geometry varied several other parameters. These primarily show an 1/ d scaling between the lateral beam–electrode distance d (see Fig. 1b ) and the capacitance change per nanometre beam displacement, as expected for a capacitive interaction. As the beams tend to stick to the side electrodes at very low gap sizes, the fabrication of smaller defect-free gaps by conventional scanning electron microscopy lithography and dry and wet etching was not successful. We have investigated devices with gap widths varying between 110 nm and 60 nm. Supplementary Figure S2 shows the coupling strength (black squares) extracted from the quality factor versus microwave frequency curves, as shown in Fig. 3b , for different values of d . The dotted red curve depicts the capacitance gradients obtained from the simulation multiplied with a scaling factor to fit the measured coupling strength. The dependence of the coupling strength on the gap size in the measurements is qualitatively reproduced by the simulations. How to cite this article: Faust, T. et al . Microwave cavity-enhanced transduction for plug and play nanomechanics at room temperature. Nat. Commun. 3:728 doi: 10.1038/ncomms1723 (2012).